The critical power to maintain thermally stable molecular junctions With the rise of atomic-scale devices such as molecular electronics and scanning probe microscopies, energy transport processes through molecular junctions have attracted notable research interest recently. In this work, heat dissipation and transport across diamond/benzene/diamond molecular junctions are explored by performing atomistic simulations. We identify the critical power P cr to maintain thermal stability of the junction through efficient dissipation of local heat. We also find that the molecule–probe contact features a power-dependent interfacial thermal resistance R K in the order of 10 9 kW −1 . Moreover, both P cr and R K display explicit dependence on atomic structures of the junction, force and temperature. For instance, P cr can be elevated in multiple-molecule junctions, and streching the junction enhances R K by a factor of 2. The applications of these findings in molecular electronics and scanning probing measurements are discussed, providing practical guidelines in their rational design. Beyond the foreseen limits of conventional silicon integrated circuits, molecular electronics has gained wide attention nowadays by holding great promises in transcending Moore’s law and pushing the limit of downsizing devices [1] . Single or multiple molecules could serve as active electronic components [2] , displaying advantages over conventional semiconductors (for example, reduced size [3] , flexibility [4] , convenience in fabrication [1] , [5] , wide material selection [1] , [3] , [6] , [7] and so on). In this scenario, molecular junctions represent the ultimate limit to the miniaturization of transistors and energy conversion devices [3] , [8] . On the other hand, the presence of interface critically defines underlying physical processes at atomic-scale, such as heat or electronic transport across the tip–sample contact in the scanning thermal microscope (SThM) [9] , [10] , scanning tunnelling microscope (STM) [11] , as well as thermoelectric energy conversion in molecular junctions [12] . Although limited by technical challenges, there are increasing activities focusing on the structural, electronic and thermal behaviours of atomic-scale junctions through experimental and theoretical approaches [12] , [13] , [14] , [15] , [16] , [17] , [18] , [19] , [20] , as well as mechanistic studies of SThM and STM [10] , [21] , [22] , [23] . For example, Huang et al. [24] probed the effective temperature of single-molecule junctions with current-induced local heating as a function of molecular length and applied bias voltage. Lee et al. [3] identified the correlation between electronic transmission characteristics of atomic-scale junctions and heat dissipation. Losego et al. [6] demonstrated a link between interfacial bonding characters and thermal conductance at the atomic level. However, the processes of heat dissipation and transport in molecular junctions still remain poorly understood [3] , [6] , [24] , [25] , [26] , [27] , which prohibits continuously growing development of aforementioned applications. In this work, we investigate heat dissipation and conduction processes through diamond/benzene/diamond junctions by performing classical molecular dynamics (MD) simulations. The atomic structures of explored systems are shown in Fig. 1a . We consider heat generation in molecular electronics with energy transferred from electrons to the nuclear motion through the electron-vibration coupling, as well as heat dissipation into thermal reservoirs it connects. The latter process balances local heating effect in the steady state (see Methods for details). We assess the thermal stability of the junction by defining a criterion for the power of heat generation P cr , below which the temperature of the molecule T M can be well maintained within a limited range from the environmental temperature T 0 . Heat transport across the junction is then quantified through the interfacial thermal resistance (ITR), or Kapitza thermal resistance R K , by considering effects of atomic structures, mechanical loads and environmental temperature as usually encountered in experimental conditions. These results are then discussed with respect to their key applications such as molecular electronics and SThM. 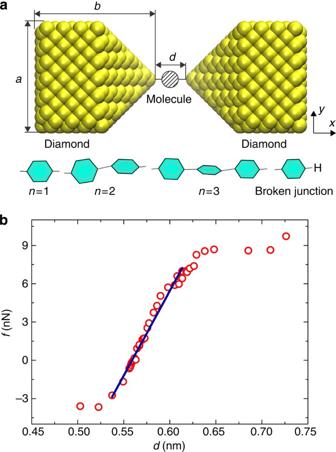Figure 1: Atomic structures of molecular junctions. (a) The diamond/benzene/diamond junction with benzene molecules covalently bonded to carbon atoms at the tips of two diamond probes. The distance between two probes isd, and the width and length of each probe area=2.05 nm andb=2.05 nm, respectively. (b) The stretching force applied to the single-molecule junction, measured as a function ofd. The results can be fitted to a linear relationf=−74.13+132.62dnN fordbetween 0.54 and 0.62 nm. Figure 1: Atomic structures of molecular junctions. ( a ) The diamond/benzene/diamond junction with benzene molecules covalently bonded to carbon atoms at the tips of two diamond probes. The distance between two probes is d , and the width and length of each probe are a =2.05 nm and b =2.05 nm, respectively. ( b ) The stretching force applied to the single-molecule junction, measured as a function of d . The results can be fitted to a linear relation f =−74.13+132.62 d nN for d between 0.54 and 0.62 nm. Full size image Heat dissipation in a single-molecule junction The atomic structure of a molecular junction depends markedly on the mechanical load it bears. Thus we first identify the load-free configuration of the junction from the relationship between the applied force ( f ) and distance ( d ) between two probes (or leads) the molecules attach to. From our MD simulation results, we find that f increases with d linearly for d ranging from 0.54 to 0.62 nm ( Fig. 1b ). The tensile stiffness of the single-molecule junction is 132.62 Nm −1 . This value is reduced as d increases beyond the linear range, where the molecule–probe contact starts to break down by rupturing bonds at the interface. The molecular junction is fully relaxed at d =0.56 nm. Based on this configuration we explore the heat dissipation process by injecting a heat flux of P , that is, we add extra kinetic energy to the degrees of freedom in the system. This procedure mimics the heat produced by Joule heating in practice due to electron–phonon and electron–electron scattering. With this local heating effect, temperature of the benzene molecule increases initially before reaching a plateau at T M within a time scale τ in the order of tens of picoseconds, which scales linearly with R K based on a diffusive resistor model [28] . In Fig. 2 , we plot T M against P and identify two characteristic profiles. At low P values, T M cannot be distinguished from the environment ( T ). We can then define a criterion for thermal stability of the molecular junction as T M − T 0 <Δ T th ( Supplementary Fig. 1 ). Specifically for a threshhold of Δ T th =50 K, we obtained a critical power of P cr =0.3 μW for the single-molecule junction. While for P > P cr , heat generation in the molecule is heavily localized and efficient thermal dissipation through the molecule–probe contact cannot be activated. 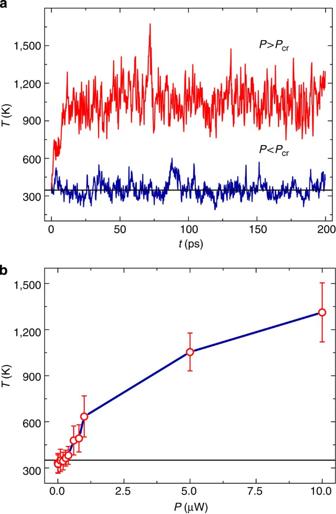Figure 2: Heat dissipation in the single-molecule junctions. (a) ,Time evolution of temperature (T) in the benzene molecule atP=5 μW (P>Pcr, the red curve) andP=0.2 μW (P<Pcr, the blue curve). The steady state of thermalization is established within a time scale of ~10 ps. HerePcris 0.3 μW for ΔTth=50 K. The black reference line indicatesT=350 K, that is, 50 K above the environmental temperature. (b)Tmeasured as a function of the heat powerP(red circles and blue lines linking them). The error bars show their standard deviations over time. Figure 2: Heat dissipation in the single-molecule junctions. ( a ) ,Time evolution of temperature ( T ) in the benzene molecule at P =5 μW ( P > P cr , the red curve) and P =0.2 μW ( P < P cr , the blue curve). The steady state of thermalization is established within a time scale of ~10 ps. Here P cr is 0.3 μW for Δ T th =50 K. The black reference line indicates T =350 K, that is, 50 K above the environmental temperature. ( b ) T measured as a function of the heat power P (red circles and blue lines linking them). The error bars show their standard deviations over time. Full size image Thermal conduction across a single-molecule junction The Kapitza resistance R K =Δ T / J is a measure of ITR. Here J is the heat flux and Δ T is the change in temperature across the molecule–probe interface. At room temperature, typical values of R K for nonbonding and covalently bonded interfaces between bulk materials are 3.33 × 10 −8 (Pb/H/C) [29] and 1.43 × 10 −9 m 2 kW −1 (TiN/Al 2 O 3 ), respectively [30] . From our heat dissipation simulation results ( Fig. 2b ), we obtain R K =Δ T / J =1.25−6.12 × 10 9 kW −1 ( J = P ) for P ranging from 10 to 0.1 μW. These values are further validated by performing non-equilibrium MD (NEMD) simulations where a temperature gradient is built up across the junction and thermal relaxation (TR) simulations where a heat pulse is introduced to drive heat transfer (see details in Methods) [31] , [32] . We obtain consistent results for the ITR from these different approaches, that is, R K =3.81 × 10 9 kW −1 from NEMD and 4.49–5.68 × 10 9 kW −1 from TR simulations, which are about one order lower than the experimental and theoretical result ( R K ~20 × 10 9 kW −1 ) for the alkane–gold junction [25] , [26] , [33] . R K depends critically on the molecular structure of junctions. We quantify the effect of structural distortion under mechanical loads by tuning the distance d between two probes. For f ranging from −4.12 to 7.2 nN, the molecular junction displays significant conformational change but no structural failure. The dependence between R K and f is summarized in Fig. 3a . The change in R K lies below 0.5 × 10 9 kW −1 for f <0 nN, and increases with f in tension ( f >0 nN). For f =7.2 nN, R K is enhanced by twofold in comparison with the value measured for the relaxed structure. The changes in R K can be explained from a structural perspective. As the junction is stretched ( f >0 nN), covalent C–C bonds at the molecule–probe contact are elongated along the direction of heat transport, while bonds in the molecule remain almost undeformed. As a consequence, frequencies of vibrational modes of the molecular junction are red-shifted. This softening effect raises the thermal resistance by reducing stiffness of the structure and thus group velocities of propagating vibrational modes [34] , [35] . When the value of d exceeds 0.65 nm ( f =9.0 nN), the molecular junction breaks at one of the molecule–probe contacts. In the broken junction ( Fig. 1a ), the ITR R K =61.38 × 10 9 kW −1 becomes one-order higher than that for unbroken ones due to the newly formed, much weaker (van der Waals) interfaces. In contrast, when the junction is compressed ( f <0), changes in all bond lengths are negligible (<0.02 Å) and structural distortion at molecule–probe contact is identified majorly as bond angle bending ( Supplementary Fig. 2 ). This explains the almost unchanged R K compared with its value at f =0. 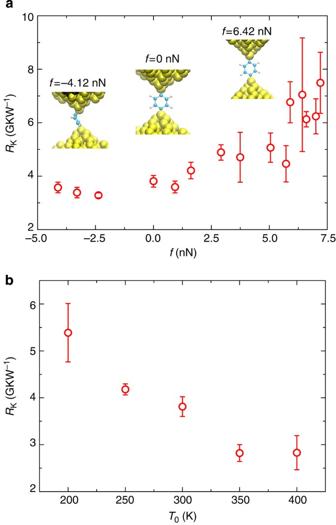Figure 3: Dependence of the interfacial thermal resistance on force and temperature. (a) The ITRRKmeasured across the single-molecule junction increases with the forcefunder tension and remains almost constant in compression. (b)RKplotted as a function of the environment temperatureT0. The error bars show standard deviations ofRKcalculated from five independent MD simulations. Figure 3: Dependence of the interfacial thermal resistance on force and temperature. ( a ) The ITR R K measured across the single-molecule junction increases with the force f under tension and remains almost constant in compression. ( b ) R K plotted as a function of the environment temperature T 0 . The error bars show standard deviations of R K calculated from five independent MD simulations. Full size image Using NEMD simulations, we further explore the dependence of R K for the single-molecule junction on the environmental temperature T 0 . The results summarized in Fig. 3b show that R K decreases with increases in T 0 , from 5.39 × 10 9 kW −1 at 200 K to 2.82 × 10 9 kW −1 at 400 K. The saturation of R K at high temperature (above 300 K) can be attributed to the radiation limit that arises from the mismatch between vibrational modes in benzene molecules and diamond [36] . This temperature dependence is similar as the one measured at a Au/SAM/Au interface [26] , but is in contradiction to crystalline materials featuring a linear T -dependence of thermal resistance at high temperature, where Umklapp processess play the critical role. Heat dissipation in a multi-molecule junction In a multiple-molecule junction, the inter-molecule coupling plays additional roles in defining the heat dissipation and transport processes. We explore this effect by studying the dependence of R K and P cr on the number of benzene molecules n in the junction. To exclude the effect of mechanical loads and temperature, all multi-molecule junctions are simulated in their relaxed configurations at 300 K. Values of ITR measured in our MD simulations are plotted as a function of n in Fig. 4 , from which we see that R K increases with n and slowly approaches a plateau, corresponding to a dominant contribution from the molecule–probe contacts. This dependence is similar as the simulation results reported for R K across multiple graphene layers between bulk silicon carbide, with weak van der Waals interfaces between them [37] . 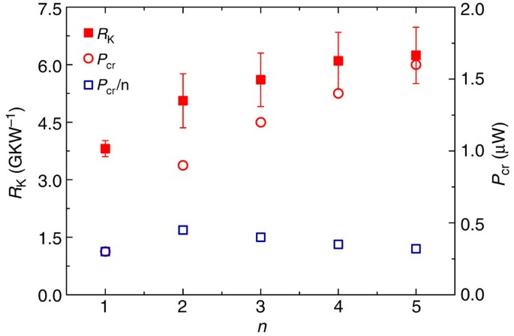Figure 4: Heat dissipation and transport in a multi-molecule junction. The ITR (RK), the critical flux power (Pcr), and the critical power per molecule (Pcr/n) plotted as a function of the number of molecules (n) in the junction. The error bars show standard deviations ofRKcalculated from five independent MD simulation. Figure 4: Heat dissipation and transport in a multi-molecule junction. The ITR ( R K ), the critical flux power ( P cr ), and the critical power per molecule ( P cr / n ) plotted as a function of the number of molecules ( n ) in the junction. The error bars show standard deviations of R K calculated from five independent MD simulation. Full size image For weakly interacting interfaces between materials, atomic structures and interaction at the contact govern heat transport processes instead of properties of the materials themselves. This can be captured in theoretical models, such as the acoustic mismatch model and diffusive mismatch model, which sets the upper and lower bounds of R K , respectively [38] . In this scenario, vibrational mode coupling across the interface governs thermal transport in a molecular junction. To gain more insights into the R K – n dependence, we plot vibrational spectra for both diamond probes and benzene molecules in Fig. 5a and Supplementary Fig. 3 . These results indicate that the spectra for different benzene molecules share common features. Thus we can consider the benzene chain as a whole unit and assume a diffusive transport mechanism across the interfaces, as illustrated in Fig. 5c [39] . We consider the junction as a serial combination of three-resistor units, where R C represents the contact resistance at the molecule–probe interface and R M is the intrinsic resistance of benzene molecules. From the calculated vibrational spectra, we find that R C is much higher than R M and the former resistance dominates the contributions to R K. We also calculate the overlap of vibrational spectra between benzene molecules and diamond probes by integrating them over the frequency range [40] . As the interfacial conductance is positively correlated with the overlap [40] , [41] , results shown in Fig. 5b indicate a significant increase of R K while n changes from 1 to 2, followed by a reduced n dependence for n >2, which explain our simulation results in Fig. 4 . 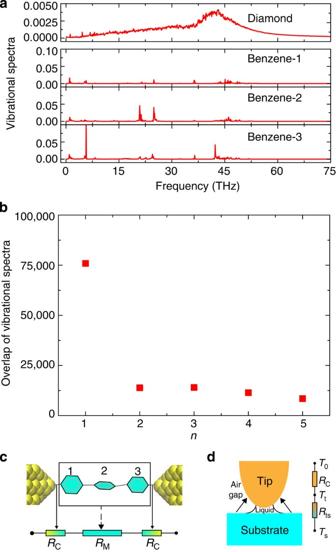Figure 5: Vibrational spectra analysis of molecular junctions. (a) Normalized local vibrational spectra in the diamond probes and benzene molecules of a three-molecule junction. (b) Overlap of the vibrational spectra in the probes and molecules plotted as a function of the number of molecules (n) in the junction. (c) A three-resistor model for the junction. (d) A schematic illustration of SThM. The parameters are explained in the text. Figure 5: Vibrational spectra analysis of molecular junctions. ( a ) Normalized local vibrational spectra in the diamond probes and benzene molecules of a three-molecule junction. ( b ) Overlap of the vibrational spectra in the probes and molecules plotted as a function of the number of molecules ( n ) in the junction. ( c ) A three-resistor model for the junction. ( d ) A schematic illustration of SThM. The parameters are explained in the text. Full size image We further characterize the critical power P cr for multiple-molecule junctions with Δ T th =50 K. The results in Fig. 4 show that P cr increases with n , as heat capacity of the junction increases with n and more heat generation could be accomodated. Considering the multiple-molecule nature in such a junction, we also plot P cr / n in Fig. 4 , which increases from n =1 to 2, followed by a slow decrease for n >2. This trend agrees with our previous discussion on the vibrational spectra in Fig. 5 , indicating a lower ITR between benzene molecules than that at the molecule–probe contact. For molecular electronics, the critical power density P cr defines its thermal stability and device performance. Hot spots could nucleate and temperature of the junction will rise significantly above the environmental temperature at P > P cr . The value P cr =0.3 μW (Δ T th =50 K) identified for the single-molecule junction corresponds to a marginal areal power density of 78.9 MW cm −2 . Here we calculate the area of junction as the size of benzene molecules, which is A =6 × 4π × d C–C 2 /4 ( d C–C is the C–C bond length). Potential breakdown of the device due to the local heating effect must be taken into account in this situation. Using multiple-molecule junctions with higher heat capacity, or adding heat sinks could help to boost the device performance. On the other hand, the value of P cr also defines the minimal Joule heating power to drive a temperature difference across the interface between molecules and probes, which enables the probe of thermal transport parameters in molecular junctions. SThM maps local temperature and thermal conductivity of materials. Its key component is the thermal probe consisting of a thermocouple junction at the end of its tip. The tip–sample interface for heat transport includes a solid contact, a thin liquid bridging film and an air gap [10] , [42] , which can be captured in a thermal resistor model as illustrated in Fig. 5d [11] . The relation between the temperature T 0 in the environment and T s , T t in the sample and tip is T t = T s +( T 0 − T s )/(1+ c ), where c = R c / R ts is the ratio between thermal resistance of the probe ( R c ) and tip–sample contact ( R ts ). From this model, one finds that changes in T s can be extracted from variations in T t as Δ T t /Δ T s = c /(1+ c ). This relation suggests that the accuracy of sample temperature measurement depends explicitly on c , which must be sufficiently high for acceptable SThM performance. The tip–sample thermal contact is similar to the single-molecule junctions explored here. Our results in Fig. 3 then indicate that when the mechanical load is zero or compressive, or the heat flux is high enough, a high value of c could be achieved. The bulk thermal conductivity of sample and the environment temperature, although could further modify heat transport at the contact, are usually constants in the measurement [39] . To assess the validity of SThM measurements, the force applied and power of heat generation should be well calibrated. The single-molecule junction we study here is non-metallic, and the electrical resistance is expected to be much higher than that of the Au/1,4-dicyanobenzene/Au junction (6.47 MΩ) [3] , [43] . Following the interfacial Wiedemann–Franz law that relates interfacial electrical conductance to its electrical thermal conductance κ e (ref. 44 ), we estimate κ e =1.14 pW K −1 , about two orders lower than κ =0.262 nW K −1 for the single-molecule junction explored here. Thus the vibrational contribution we focus on plays the major role in the thermal dissipation and transport processes across non-metallic molecule junctions. In brief, we investigate heat dissipation and transport across benzene-based molecular junctions using MD simulations. For heat dissipation in the molecular junction, we identify the critical power P cr to maintain its thermal stability, beyond which its temperature will rise above the threshold Δ T th defined for specific applications. P cr increases with the number of molecules n in the junction, and P cr / n peaks at n =2. We use the ITR R K to quantify thermal transport across the molecule junctions. The value of R K is in the order of 10 9 kW −1 , which displays power and temperature dependences. Moreover, R K can be enhanced by a factor of 2 when the junction is stretched. These findings are explained by using a simple resistor chain model and analyzed by vibrational spectra analysis. Our results are discussed on their key applications in molecular electronics and scanning probe techniques, such as SThM and STM, which provide practical design guidelines for relevant applications by offering fundamental understandings of the thermal energy transfer process. Atomic structures of molecular junctions We construct molecular junctions by covalently bonding benzene molecules and the tips of diamond probes. This setup is similar to the Au/benzenedithio/Au junctions experimentally explored recently [45] . The width and length of the probe are a =2.05 nm and b =2.05 nm ( Fig. 1 ), which are large enough to allow tracking heat transport across the junction, considering the high thermal conductivity of diamond. The force applied across the junction is obtained by relaxing the junction structure while keeping the distance d between the two probes fixed. MD simulations All MD simulations are performed using the large-scale atomic/molecular massively parallel simulator package [46] . The interatomic interactions for diamond and benzene are calculated using the adaptive intermolecular reactive empirical bond order (AIREBO) potential functions with the torsion term and van der Waals interaction included [47] . MD simulations based on AIREBO potential functions and parameters are validated to predict reasonably structural, mechanical and thermal properties of hydrocarbon system [48] . The time step for equation-of-motion integration is set to 0.2 fs to assure energy conservation in the absence of thermostat coupling. Open boundary conditions are used in all three dimensions. We simulate the heat dissipation process by scaling atomic velocities in the molecular junction. Temperature in two 0.5 nm-thick slabs at the ends of both diamond probes is maintained at 300 K. To confirm that the classical MD simulations yield a reliable description of the thermal dissipation and transport processes, we compare vibrational spectra of the molecular junction calculated from classical and quantum MD simulations implemented through the path-integral formula [49] . The vibrational spectrum in a finite-temperature simulation is calculated as the Fourier transform of velocity auto-correlation functions. Compared with the vibrational density of states obtained by diagonalizing the dynamical matrix, the vibrational spectrum shows the population of these states, that is, the vibrational modes. The results ( Supplementary Fig. 4 ) show that within the temperature range explored in this work, the consistence between these two approaches is very well preserved. In analysing the temperature distribution, we track the temperature in the benzene molecules and the diamond probes by averaging temporally at a time inteval of 2 ps, spatially within 0.1 nm-thick bins along the junction ( x -direction in Fig. 1 ). In TR simulations, we extract the relaxation time τ after applying a 2 ps heat pulse and calculate R K using R K =2 τ / C , where C =135.69 J K −1 mol −1 is the heat capacity of liquid benzene at room temperature [50] . The Kapitza resistance R K is also calculated in NEMD [26] . We first equilibrate the diamond–benzene–diamond hybrid using a Nosé–Hoover thermostat at 300 K for 200 ps. The system is then further relaxed in a constant atom number-volume-energy (NVE) ensemble for 50 ps before the heat flux is pumped into diamond probes, which simulate the heat source and sink. The temperature of two 0.5-nm-thick slabs in the diamond probes is controlled to be 350 K and 250 K, respectively, using a Berendsen thermostat. We track temperature evolution in the junction and calculate the thermal flux J along the thermal gradient by summing energy in/out flow in the thermal probes. The ITR is then evaluated by following Kapitza’s definition, that is, R K =Δ T / J , where Δ T is the temperature difference across the interface. How to cite this article: Wang, Y. and Xu, Z. The critical power to maintain thermally stable molecular junctions. Nat. Commun. 5:4297 doi: 10.1038/ncomms5297 (2014).